Using carbon dioxide as a building block in organic synthesis A more sensible resource management is the prerequisite for the sustainable development of future generations. However, when dealing with the feedstock of the chemical industry, the level of sustainability is still far from satisfactory. Until now, the vast majority of carbon resources are based on crude oil, natural gas and coal. In addition to biomass, CO 2 offers the possibility to create a renewable carbon economy. Since pre-industrial times, the amount of CO 2 has steadily increased and nowadays CO 2 is a component of greenhouse gases, which are primarily responsible for the rise in atmospheric temperature and probably abnormal changes in the global climate. This increase in CO 2 concentration is largely due to the combustion of fossil fuels, which are required to meet the world’s energy demand [1] . Obviously, there is an urgent need to control CO 2 emissions and develop efficient carbon capture systems. Although the extensive use of carbon dioxide for chemical production cannot solve this problem alone, CO 2 is a useful one-carbon (C1) building block in organic synthesis due to its abundance, availability, nontoxicity and recyclability. As a result, valorization of CO 2 is currently receiving considerable and ever increasing attention by the scientific community [2] , [3] , [4] . However, activation and utilization of CO 2 is still problematic due to the fact that it is the most oxidized form of carbon, which is also thermodynamically stable and/or kinetically inert in certain desired transformations. Consequently, most of the known studies used highly reactive substrates and/or severe reaction conditions to activate CO 2 , limiting the application of such methods. In particular, the catalytic coupling of CO 2 with energy-rich substrates, such as epoxides and aziridines, to generate polycarbonates/polycarbamates and/or cyclic carbonates/carbamates has drawn significant attention over the past decades. To create C-C bonds with CO 2 , the use of carbon nucleophiles is specifically limited to strong nucleophilic organolithiums and Grignard reagents, as well as phenolates. Along with the rapid development of organometallic chemistry and catalysis (see Box 1 ), various types of efficient CO 2 transformations in organic synthesis have been discovered in the past decades, greatly improving its efficiency and applicability. This review will describe the most recent advances made in the area of CO 2 valorization—turning CO 2 into a useful chemical feedstock—under mild conditions. A special focus is given on the reaction modes for the CO 2 activation and its application as C1 building block in organic synthesis. While classical methods for CO 2 hydrogenation have been reviewed elsewhere and will not be included here [5] , [6] , [7] , the following subjects will be addressed: (1) novel transformations using carbon dioxide (briefly summarized in Fig. 1 ); (2) different reaction modes for CO 2 activation (main focus of this review); and (3) potential new applications of CO 2 valorization. 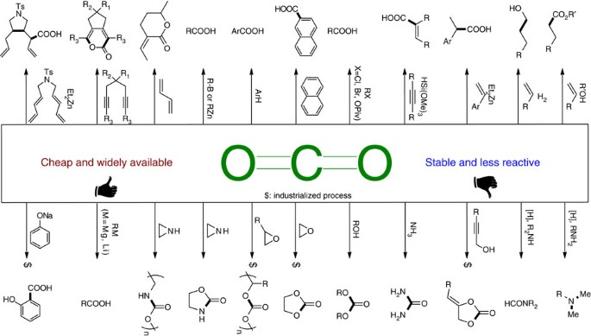Figure 1: Representative examples using CO2as C1 building block in organic synthesis. Along with the rapid development of organometallic chemistry and catalysis, various types of efficient CO2transformations were have been discovered in the past decades. However, in general, the substrates’ scope and efficiency of these reactions are still limited due to the requirement of reactive agents for CO2activation. As a result, only a few processes have been industrialized until now (marked by $). Figure 1: Representative examples using CO 2 as C1 building block in organic synthesis. Along with the rapid development of organometallic chemistry and catalysis, various types of efficient CO 2 transformations were have been discovered in the past decades. However, in general, the substrates’ scope and efficiency of these reactions are still limited due to the requirement of reactive agents for CO 2 activation. As a result, only a few processes have been industrialized until now (marked by $). Full size image Box 1: Coordination modes of CO 2 with transition metals. A key issue for valorization of CO 2 to valuable chemical intermediates and further on to consumer products relies on efficient catalysts. As a basis, an insightful understanding of the detailed organometallic chemistry of CO 2 is of great importance for the further design of the catalytic processes. In fact, the chelating mode between transition metal centres and CO 2 has been investigated intensively via stoichiometric experimental studies [46] , [47] . As shown above, CO 2 has multiple reactive sites: the carbon atom is an electrophilic Lewis acid centre and the oxygen atoms act as weak nucleophilic Lewis base. In its ground state, carbon dioxide possesses two equivalent C-O bonds that could both coordinate to a transition metal centre. As a result, a series of transition metal CO 2 complexes are known. If a metal centre reacts with one molecule of CO 2 , there are five different chelating modes possible. More specifically, complex I with an M-C bond is sometimes termed as a metallacarboxylate. Electron-rich metal centres are more feasible to form these types of complexes via electron transfer from metal centre to carbon atom. Adduct II (end-on type) seems less plausible due to the weak interaction between the lone pair of only one oxygen atom and the metal centre. Meanwhile, complex III should be more stable, since CO 2 acts as a bidentate ligand with two oxygen atoms. In this case, a more electron-deficient metal centre is favoured for the electron transfer from oxygen atom to transition metal. A combination of the above two mentioned electron transfer processed affords the three-membered metallacycle complex IV . Moreover, the side-on-bonding π-complex V can also be formed in a similar spatial arrangement of atoms through the coordination of the C-O double bond to the central metal. On the basis of these different coordination and activation modes, well-designed transition metal complex catalysts are able to promote the reactivity and also control the selectivity of CO 2 fixation reactions in the organic synthesis. This promising research area still has many novelties to be discovered. Activation modes for catalytic valorization of CO 2 CO 2 is the most stable form of oxidized carbon compounds. Nevertheless, it reacts easily with strong nucleophiles to form new C-C or C-H bonds. However, to use carbon dioxide in a more benign and practical manner, efficient transformations with less-activated substrates under mild conditions have to be developed. Obviously, reactions of CO 2 that require a high-energy input are not benign because in general this energy leads also to formation of CO 2 . Cooperative effects for CO 2 activation To achieve low-energy-demanding synthetic protocols using CO 2 as C1 building block, efficient interactions with the specific substrate is required. In this respect, cooperative activation of carbon dioxide with such substrates often in the presence of a suitable catalyst is of fundamental importance. Among the CO 2 functionalization methodologies, traditional examples that make use of cooperative effects are the catalytic valorization of energy-rich substrates (for example, strong nucleophilic organometallic reagents, epoxides, aziridines and so on). They provide a straightforward way for the thermodynamic driving force. One of the more successful processes for CO 2 utilization for material synthesis is the catalytic productions of cyclic carbonates and polycarbonates from epoxides [8] , which has been industrialized as well [9] . Nowadays, cyclic carbonates are widely used as organic synthetic intermediates, aprotic polar solvents, precursors for biomedical applications and raw materials for engineering plastics. Although this 100% atom economical reaction has been commercialized for the synthesis of ethylene and propylene carbonates for over 50 years [10] , recently a variety of highly selective and reactive catalysts were developed. Representative systems are summarized in Fig. 2 (ref. 11 ). Notably, in 1983, Inoue and co-workers described in their seminal work that a (TPP)AlOMe complex can trap carbon dioxide readily and reversibly at room temperature. The trapped carbon dioxide is active enough to react with epoxide at ambient conditions to afford the corresponding cyclic carbonates [12] . Since then, various metalloprophyrin catalysts were studied in this transformation. For example, in 2007, Jing et al. [13] reported a Co(TPP)(OAc)/PTAT (phenyltrimethylammonium tribromide) catalyst system to achieve this CO 2 fixation at room temperature and low pressure. More recently, Sakai et al. developed a highly active bifunctional porphyrin catalyst, which combines an organocatalytic group (quaternary ammonium bromide) and a metal ion (Mg II ). It shows a high turnover number (TON=103,000) for the synthesis of cyclic carbonates from CO 2 and epoxides under solvent-free conditions [14] . Related salen-based complexes represent another kind of effective catalysts for the electrophilic addition of CO 2 to epoxides. Already in 2001, air stable and commercially available Cr(III) salen complexes were presented to be highly efficient catalysts in the coupling of carbon dioxide with epoxides at mild temperatures and pressures by the group of Nguyen [15] . While most of the work in this area made use of pressurized carbon dioxide, Kleij and co-workers [16] showed that inexpensive and structurally simple Zn(salphen) catalysts can be employed as efficient catalysts for the synthesis of cyclic carbonates from CO 2 and terminal epoxides under mild conditions (2 bar CO 2 ). Noteworthy, the group of North [17] communicated the formation of cyclic carbonates even at 25 °C and 1 bar CO 2 using bimetallic Al III -salen complexes. More recently, the Kleij group [18] presented an easily accessible amino triphenolate complex based on Al III metal centre. This complex is demonstrated to be a highly active and versatile catalyst for organic carbonate formation. Remarkably, initial turnover frequencies as high as 36,000 per hour during the cycloaddition of CO 2 to epoxides were obtained with TONs exceeding 100,000. Except for the above-mentioned sophisticated metal complexes, simple onium salts can also acts as efficient catalysts. For instance, a combination of ZnCl 2 and [Bmim]Br reported by Xia’s group [19] is a really practical, highly efficient and environmentally benign catalyst system for the chemical fixation of CO 2 with epoxides. Finally, it is worth mentioning that Jiang, Han and co-workers [20] in 2011 found that cellulose/KI was a very active, selective and recyclable catalyst for this reaction without the assistance of any transition metal catalyst. 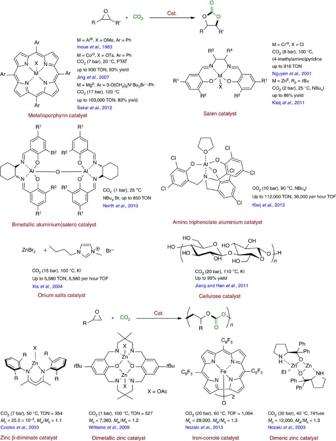Figure 2: Established catalysts and reaction conditions for the catalytic productions of cyclic carbonate and polycarbonate from oxiranes using CO2as the feedstock. Examples include metalloporphyrin, salen, metal-corrole, dimetallic as well as metal-free catalysts. Figure 2: Established catalysts and reaction conditions for the catalytic productions of cyclic carbonate and polycarbonate from oxiranes using CO 2 as the feedstock. Examples include metalloporphyrin, salen, metal-corrole, dimetallic as well as metal-free catalysts. Full size image The direct polymerization of epoxides with CO 2 to produce polycarbonates has been accomplished too. In this respect, the contributions from Coates and co-workers [21] , [22] described very active zinc β-diiminate catalysts for the synthesis of monodispersed, highly alternating carbon dioxide/epoxide copolymers with high molecular weight. In addition, the group of Williams [23] demonstrated a zinc-based macrocyclic bimetallic catalyst for epoxide/CO 2 copolymerization, which shows remarkable activity at only 1 bar of CO 2 . Very recently, iron−corrole complexes were synthesized by Nozaki and co-workers [24] to copolymerize epoxides with CO 2 , providing the first example of iron-catalysed PO (propylene oxide)/CO 2 and GPE (glycidyl phenyl ether)/CO 2 copolymerization. The same group also demonstrated the stereoselective alternating copolymerization of cyclohexene oxide and CO 2 with dimeric zinc complexes for the first time [25] . Besides, improved catalysts are still desirable to better control the properties of the resulting materials [26] . Similarly, many efforts are also devoted to designing catalysts able to promote the reaction of CO 2 with less-reactive oxiranes, which could also provide novel materials [27] . Apart from the utilization of energy-rich substrates (for example, epoxides), catalytic reductive formylation and methylation of amines represent important modern examples for cooperative effects in the activation of CO 2 . Here the activation energy for reductive deoxygenation of CO 2 is significantly decreased by the coordination of amines to CO 2 and the formation of N-C bonds (in a carbamate or urethane intermediate), which thus facilitates the reduction of CO 2 . Likely, the other advantage of amines is to increase CO 2 concentration in the condensed phase [28] . These transformations represent diagonal approaches to the chemical recycling of CO 2 , which combine both reduction of CO 2 and C-N bond formation processes ( Fig. 3 ) [29] . More specifically, Cantat and co-workers reported an unprecedented organocatalytic synthesis of formamides from CO 2 . Mechanistic studies uncovered the synergistic effect of the organocatalyst TBD (triazabicyclodecene) and amine substrates in the promotion of CO 2 activation ( Fig. 3 , equation a) [30] . Shortly afterwards, a highly active N -heterocyclic carbene organocatalyst was designed by the same group for the formylation of N-H bonds in various amines and heterocycles under very mild conditions using CO 2 and polymethylhydrosiloxane (PMHS; Fig. 3 , equation b) [31] . 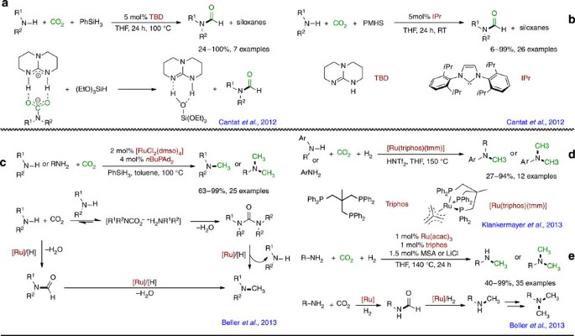Figure 3: Catalytic reductive formylation and methylation of amines with CO2as C1 source. (a,b) Organocatalytic formylation of amines with CO2using silanes as the reductants. (c) Ru-catalysed methylation of amines with CO2using silanes as the reductants. (d,e) Ru-catalysed methylation of amines with CO2using H2as the reductant. Figure 3: Catalytic reductive formylation and methylation of amines with CO 2 as C1 source. ( a , b ) Organocatalytic formylation of amines with CO 2 using silanes as the reductants. ( c ) Ru-catalysed methylation of amines with CO 2 using silanes as the reductants. ( d , e ) Ru-catalysed methylation of amines with CO 2 using H 2 as the reductant. Full size image Meanwhile, the methylation of amines via six-electron reduction of CO 2 remains unknown until 2013. The market value of methylamines such as MeNH 2 , Me 2 NH and Me 3 N exceeds 4,000 Euro per ton. Therefore, the reductive methylation of amines with CO 2 can create additional value. In early 2013, our group developed a Ru catalyst system that was able to convert carbon dioxide and amines into various kinds of N -methylated products in the presence of hydrosilanes (PhSiH 3 ). Notably, diverse functional groups were well tolerated under these conditions ( Fig. 3 , equation c) [32] . In the same year, Cantat et al. [33] reported zinc catalysts able to perform the methylation of amines with CO 2 and hydrosilanes at low pressure. Furthermore, the selective reduction of ureas was possible under similar reaction conditions. Although some silanes are considered to be waste products of the silicone industry, all these methodologies are limited by the accessibility of the hydrosilanes and an additional workup step to remove siloxane by-products. Obviously, catalytic methylations using CO 2 and H 2 represent a greener method with H 2 O as the only by-product. In this respect, two research groups independently reported similar catalytic systems shortly afterwards to convert amines into methylamines in the presence of CO 2 and H 2 . On one hand, Klankermayer and co-workers [34] presented the use of a molecularly defined ruthenium complex [Ru(triphos)(tmm)] together with readily available organic acids as co-catalysts to afford the methylation of aryl amines in good yields ( Fig. 3 , equation d). Meanwhile, the group of Beller demonstrated the efficient N -methylation of both aromatic and aliphatic amines using CO 2 /H 2 as the methylation reagent. Applying an in situ combination of Ru(acac) 3 , triphos and either acid additives or LiCl, the desired methylated amines were obtained with high efficiency. Notably, selective monomethylation of primary amines as well as the methylation of more challenging aliphatic amines proceeded smoothly under these conditions ( Fig. 3 , equation e) [35] . Interestingly, Shi et al. [36] described in 2014 heterogeneous copper catalysts for the same transformation with CO 2 and H 2 . In general, formamides are the common reaction intermediates for the above-mentioned methylation reactions. Again, this indicates the advantageous activation effect of amine substrates for the CO 2 reduction step. CO 2 fixation via oxidative cyclometallation Pioneered by the synthesis and isolation of Aresta’s complex [Ni(CO 2 )(PCy 3 ) 2 ] in 1975 (ref. 37 ), the development of low-valent metal (nickel or palladium) complexes that mediate the oxidative couplings of CO 2 with various unsaturated hydrocarbons provides a facile approach to overcome the obstacles of CO 2 fixation. While it permitted the use of CO 2 under atmospheric pressure, stoichiometric amounts of metal were necessary to generate various metallacycle complexes via the oxidative cyclometallation of Ni(0) complexes with CO 2 and olefins or alkynes ( Fig. 4 , equations a and b) [38] , [39] . The nickel-mediated stoichiometric fixation of carbon dioxide with alkenes [40] has been known for over 20 years largely due to the works from Hoberg and co-workers. However, the limited substrate scope and/or relatively harsh conditions still remain concerns for this CO 2 activation strategy. Meanwhile, only a few catalytic systems based on this strategy have been developed. In 2002, Louie et al. [41] communicated an efficient nickel-catalysed [2+2+2] cycloaddition of CO 2 and diynes in the presence of catalytic amounts of Ni(0) and specific carbene ligands ( Fig. 4 , equation c). In the same year, the group of Mori [42] , [43] developed a nickel-catalysed regio- and stereoselective ring-closing carboxylation of bis-1,3-dienes, which proceeds via insertion of CO 2 into a bis-π-allylnickel intermediate followed by a transmetalation process of the resulting cyclic nickel carboxylate with a sensitive dialkylzinc reagent ( Fig. 4 , equation d). Except for nickel-catalysed cyclization reactions, the Pd-catalysed telomerization of 1,3-butadiene with CO 2 is one of the first successful examples of the catalytic formation of a new C-C bond between CO 2 and an organic compound. Thirty years ago, Behr et al. found that the cyclization product is selectively produced employing Pd(acac) 3 and P i Pr 3 as the catalyst. The resulting δ-lactone is formed via an allylic palladium carboxylate complex as a key intermediate ( Fig. 4 , equation e) [44] . Generally, the CO 2 transformations via oxidative cyclometallation pathways are restricted to substrates with extensive π systems (for example, dienes and diynes). Interestingly, in 2008, the group of Dong discovered that Aresta’s complex catalysed the cross-coupling of organozinc reagents with CO 2 . By replacing nickel catalysts with palladium, the latter complexes were found to be catalytically active as well for the reaction of aryl zinc bromides ( Fig. 4 , equation f). The proposed mechanism consisted of an oxidative addition of Ni(0) to CO 2 to generate Aresta’s complex; transmetalation with the organozinc reagent and reductive elimination affording the corresponding zinc carboxylate that was finally hydrolysed by acidic workup ( Fig. 4 , equation g) [45] . 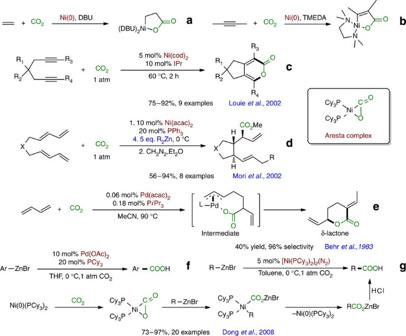Figure 4: Catalytic CO2fixation via oxidative cyclometallation with low-valent Ni and Pd complexes. (a,b) The generation of metallacycle complexes via the oxidative cyclometallation of Ni(0) complexes with CO2and unsaturated bonds. (c) Ni-catalysed [2+2+2] cycloaddition of CO2and diynes. (e) Pd-catalysed telomerization of 1,3-butadiene with CO2. (f,g) Aresta’s complex catalysed the carboxylation of organozinc reagents with CO2. Figure 4: Catalytic CO 2 fixation via oxidative cyclometallation with low-valent Ni and Pd complexes. ( a , b ) The generation of metallacycle complexes via the oxidative cyclometallation of Ni(0) complexes with CO 2 and unsaturated bonds. ( c ) Ni-catalysed [2+2+2] cycloaddition of CO 2 and diynes. ( e ) Pd-catalysed telomerization of 1,3-butadiene with CO 2 . ( f , g ) Aresta’s complex catalysed the carboxylation of organozinc reagents with CO 2 . Full size image Carboxylation reactions via CO 2 insertion into C-M bonds The formation of a thermodynamically and kinetically stable C-C bond is the most desirable form of CO 2 fixation. Since carbon dioxide is an inert electrophile, highly reactive organolithium and Grignard reagents are typically utilized as strong nucleophiles to react with CO 2 directly to construct C-C bonds and furnish valuable carboxylic acids and their derivatives. In fact, the current industrial synthesis of salicylic acid derivatives is a prime example for this type of reaction. In general, nitrogen or oxygen nucleophiles exhibit much better reactivity than carbon nucleophiles for CO 2 activation. As a result, catalytic C-C bond formation using CO 2 as C1 building block with less-reactive substrates has been and constitutes still a major challenging task for organic synthesis and catalysis research [46] . This goal can be achieved with the aid of transition metal catalysts that lower the activation energy and thus considerably increase the reaction rate for the C-C bond-forming step. Particularly, the CO 2 insertion reactions into various C-M bonds to form carboxylato complex via the formation of a new C-C bond are well known [47] . Moreover, transition metal complexes can react with less-nucleophilic organometallic reagents, for example, organoboron compounds, as well as organohalides, unsaturated bonds even activated C-H bonds to form C-M bonds efficiently, similar to their performance in the classic cross-coupling reactions [48] . Furthermore, the CO 2 insertion intermediate (RCOO-M) might be quenched in a suitable way to regenerate the catalytically active species. This provides numerous possibilities for catalytic carboxylation reactions with all the above-mentioned substrates [49] , [50] , [51] , [52] . Representative examples for such processes are listed in Table 1 including a summary of substrates, catalyst precursors, ligands, additives as well as other conditions. In addition, a comparison of the postulated mechanisms for carboxylation and hydro(bora)carboxylation reactions are presented in Fig. 5 . Table 1 A summary of carboxylation reactions of C-B, C-X and C-H bonds with CO 2 : catalytic systems and reaction conditions. 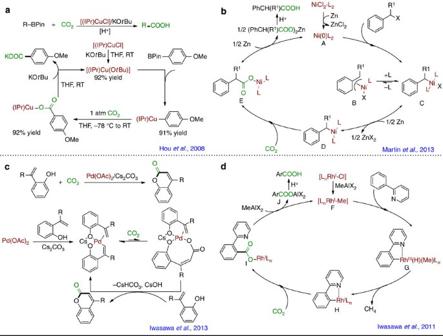Figure 5: Possible reaction mechanisms for typical carboxylation reactions with CO2. (a) Reaction mechanism for Cu-catalysed carboxylation reactions of organoboron compounds. (b) Reaction mechanism for Ni-catalysed carboxylation reactions of benzyl halides. (c,d) Directing group-assisted carboxylation of C-H bonds. Full size table Figure 5: Possible reaction mechanisms for typical carboxylation reactions with CO 2 . ( a ) Reaction mechanism for Cu-catalysed carboxylation reactions of organoboron compounds. ( b ) Reaction mechanism for Ni-catalysed carboxylation reactions of benzyl halides. ( c , d ) Directing group-assisted carboxylation of C-H bonds. Full size image Pioneered by the work of Iwasawa et al. in 2006 ( Table 1 , entry 1) the catalytic carboxylation of organoboron reagents with CO 2 in the presence of Rh [53] , Cu [54] , [55] , [56] , [57] and Ag ( Table 1 , entry 4) [58] catalysts has been developed. These coupling reagents exhibit milder nucleophilicity, better stability to air and moisture as well as higher compatibility with sensitive functional groups. Among these results, the combination of IPrCu-NHC complex and alkoxide base (M′OR′) developed by the group of Hou [55] , [57] since 2008 was found to be the most active catalyst system for the carboxylation of aryl-, alkenyl- and also alkylboronic acid derivatives ( Table 1 , entries 3 and 6). A general synthesis of various carboxylic acids with CO 2 was accomplished, and a wide range of functional groups were well tolerated. On the basis of stoichiometric experiments (taken the reactions of ArBPin, for example, as shown in Fig. 5a ), a general mechanism for such reactions was also proposed: the metathesis reaction between [(IPr)CuCl] and alkoxide generates the corresponding alkoxide complex [(IPr)Cu(OR′)], which could coordinate with organoboron reagents (R-BX 2 ) through interaction between the alkoxy group and the boron atom. Subsequent transmetalation to the copper atom generates the organocopper complex [(IPr)CuR]. Then, CO 2 insertion into the C-Cu bond yields the carboxylate [(IPr)Cu(OCOR)], which on metathesis with alkoxide base M′OR′ regenerates [(IPr)Cu(OR′)] and releases the carboxylate salt RCO 2 M′. Finally, the latter yields the carboxylic acid RCO 2 H via hydrolysis. Some key reaction intermediates, such as the copper(I) alkoxide complexes [(IPr)Cu-(OR′)], organocopper species [(IPr)CuR] and the carboxylate copper intermediates [(IPr)Cu(OCOR)], were successfully isolated and structurally characterized, which were also confirmed to be catalytically active species in these transformations. Apart from organoboron reagents, acidic C-H bonds can also undergo deprotonative metallation with specific transition metal complexes to form C-M bonds with the assistance of strong bases. Accordingly, the catalytic carboxylation of terminal alkynes ( Table 1 , entries 7–10) [59] , [60] , [61] , [62] and electron-deficient (hetero)arenes ( Table 1 , entries 11–14) [63] , [64] , [65] , [66] (pKa(C-H)<32.5) is achieved through the following CO 2 insertion and metathesis of metal carboxylate intermediates with base. Except the active copper and gold N -heterocyclic carbene complexes, Cu(diPhPhen)(PPh 3 ) 2 NO 3 ( Table 1 , entry 7) and AgI ( Table 1 , entry 9) were also demonstrated to be the effectual catalysts for the carboxylation of terminal alkynes by the group of Goossen [62] and Lu [59] , respectively. Interestingly, at higher temperature (>120 °C), the Cs 2 CO 3 -mediated carboxylation of heteroarenes ( Table 1 , entry 14) [64] and terminal alkynes ( Table 1 , entry 10) [60] with CO 2 were reported by Hu and Zhang’s groups independently as well. Later on, the group of Iwasawa showed the formation of C-M bonds by a directing group-assisted C-H activation process, which was used for subsequent carboxylation reactions with CO 2 . In fact, treatment of 2-hydroxystyrenes bearing a hydroxy group as the chelating group with catalytic amount of Pd(OAc) 2 in the presence of Cs 2 CO 3 and CO 2 afforded the corresponding coumarins via carboxylation/condensation ( Fig. 5c ) [67] . It is proposed that first the six-membered alkenyl palladium intermediate is generated by chelation-assisted alkenyl C-H bond cleavage of 2-hydroxystyrene with Pd(OAc) 2 along with coordination of the second molecule of substrate. Subsequently, the alkenyl palladium(II) species undergoes nucleophilic carboxylation to afford a palladium carboxylate intermediate, which reacts with 2-hydroxystyrene and base to give lactone with regeneration of the cyclometalated intermediate. The same group also reported another approach for the direct carboxylation reaction of aromatic C-H bonds: namely, the Rh(I)-catalysed carboxylation of aromatic compounds via chelation-assisted ortho-metalation ( Fig. 5d ) [68] . The key intermediate is proposed to be the methylrhodium(I) complex F , which undergoes chelation-assisted oxidative addition with a suitable C-H bond to afford rhodium(III) complex G , followed by reductive elimination of methane to give the nucleophilic arylrhodium(I) complex H . Consequently, nucleophilic carboxylation of intermediate H affords rhodium carboxylate I , which undergoes transmetalation with a methylaluminium reagent to give aluminium carboxylate J and regenerate the active methylrhodium(I) complex F . The oxidative addition of organo(pseudo)halides with low-valent transition metals constitutes another way to form C-M bonds. In this respect, in 2009, Martin and co-workers [69] presented a palladium-catalysed direct carboxylation of aryl bromides with CO 2 ( Table 1 , entry 15). In contrast to the reactions vide supra, this is the first example for carboxylation reactions of electrophiles instead of nucleophiles. Therefore, additional reductant (here Et 2 Zn) is needed to regenerate the catalytically active low-valent Pd(0) species. After Martin’s work, Tsuji and co-workers found that less-expensive nickel catalysts are active in carboxylation of aryl chlorides and vinyl chlorides. Notably, these reactions proceed under 1 atm CO 2 pressure at room temperature ( Table 1 , entry 16) [70] . The Ni(I) species was involved in the catalytic cycle with the aid of the Mn/Et 4 NI system as an efficient reducing agent. Although the carboxylation of aryl bromides and chlorides with CO 2 provides a straightforward synthetic route to functionalized benzoic acids, these protocols cannot be utilized to access aliphatic electrophiles, for example, for the synthesis of biologically active phenylacetic acid derivatives. Hence, it was interesting when Martin’s group reported in 2013 the first catalytic carboxylation of primary, secondary and tertiary benzyl halides utilizing CO 2 . Their protocol provides an opportunity to prepare phenylacetic acids from commercially available and cheap starting materials ( Table 1 , entry 17) [71] . The proposed catalytic cycle starts with an initial reduction of the Ni(II) pre-catalyst by Zn followed by oxidative addition to the corresponding alkyl halides, thus delivering η 3 - and η 1 -bound nickel complexes B and C in a rapid equilibrium. Generation of the reduced Ni(I) species D by Zn and CO 2 insertion affords the carboxylate nickel intermediate E . Further treatment with Zn regenerates the active Ni(0)L 2 A species and provides zinc carboxylate, which on hydrolysis delivers the final product ( Fig. 5b ). Very recently, the same group reported a novel Ni-catalysed carboxylation of aryl esters with less-activated C-O bonds ( Table 1 , entry 18) [72] . This new protocol deals with the development of a synergistic activation of CO 2 and a rather challenging activation of inert C(sp 2 )−O and C(sp 3 )−O bonds derived from simple and cheap alcohols. In general, all these modern transformations have to be compared with the classic carboxylation of Grignard reagents. The main advantage of these recent methodologies can be the tolerance of functional groups, and thus the possibility to synthesize complex carboxylic acid derivatives. On the other hand, the major drawback of all carboxylation reactions of electrophiles is the necessity to use (over)stoichiometric amounts of metals as reducing agents. Obviously, hydrogen would be a much more favourable reductant for such processes; however, no efficient regeneration of the active low-valent metal complexes have been realized yet. Significant advancements were made in the catalytic CO 2 hydrocarboxylation of unsaturated C-C bonds too. For example, in 2008, Iwasawa and co-workers reported the hydrocarboxylation of allenes and 1,3-dienes with a silyl pincer-type palladium complex. The reactions were carried out at room temperature under 1 atm CO 2 and enabled the facile and regioselective synthesis of β,γ-unsaturated carboxylic acids [73] . The reaction is believed to start with generation of a silyl pincer-type palladium hydride complex via transmetalation of AlEt 3 to (PSiP)PdOTf followed by β-hydride elimination. Hydrometalation of 1,1-disubstituted allenes preferentially afford the less-congested σ-allylpalladium intermediate, which then undergoes nucleophilic addition to CO 2 at the γ-position of the palladium regioselectively to give the carboxylate palladium complex. Finally, a transmetalation/β-hydride elimination sequence regenerates the catalytically active palladium hydride species and releases the carboxylation product as its Al salt ( Fig. 6a ). Meanwhile, the first direct hydrocarboxylation of alkenes occurred in similar manner. Rovis and co-workers [74] developed a Ni-catalysed hydrocarboxylation of styrenes using Et 2 Zn as the hydride donor with CO 2 ( Fig. 6b ). The suggested mechanism involved a nickel hydride complex as active catalyst. Afterwards, a highly regio- and stereoselective three-component Ni-catalysed syn-hydrocarboxylation of alkynes with Et 2 Zn and CO 2 using Ni(cod) 2 as catalyst and CsF as additive was presented by Ma and co-workers [75] . Although these three examples demonstrate interesting carboxylation reactions, strong and extremely air-sensitive reducing agents are indispensable. This problem is partially avoided in the copper-catalysed hydrocarboxylation of alkynes with CO 2 using hydrosilanes as milder reducing agent realized by Tsuji and co-workers ( Fig. 6c ) [76] . The fundamental catalytic steps in their hydrocarboxylation were examined by stoichiometric reactions. Treatment of the catalyst precursor [Cl 2 IPrCuF] with silane led to the catalytically active copper hydride species. It reacted with an alkyne substrate smoothly to afford the corresponding copper alkenyl complex, which on CO 2 insertion affords the copper carboxylato complex. δ-bond metathesis of this species with hydrosilane regenerated [Cl 2 IPrCuH] and provided the corresponding silyl ester. In analogy to hydrocarboxylations, catalytic boracarboxylations of alkynes with diborane and CO 2 using an N -heterocyclic carbene copper catalyst were recognized by Hou in 2012 (ref. 77 ). The reaction of [(NHC)Cu(OR)] with B 2 (pin) 2 instantly gave the borylcopper complex [(NHC)CuB(pin)]. Its subsequent reaction with internal alkyne afforded a β-boryl alkenyl complex, which undergoes the following CO 2 insertion and metathesis processes to furnish the final product ( Fig. 6d ). 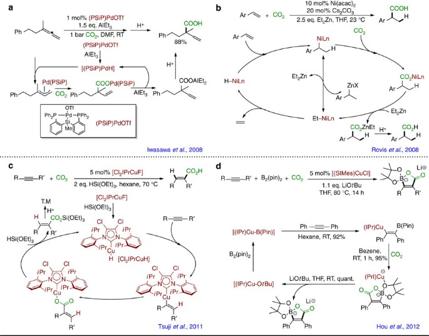Figure 6: Selected examples for hydro(bora)carboxylation reactions of alkenes and alkynes with CO2. Examples include (a) allenes, (b) styrenes and (c,d) internal alkynes. Figure 6: Selected examples for hydro(bora)carboxylation reactions of alkenes and alkynes with CO 2 . Examples include ( a ) allenes, ( b ) styrenes and ( c , d ) internal alkynes. Full size image Carbonylation reactions using CO 2 as CO surrogates Compared with all above strategies to directly use CO 2 as C1 building block in chemical synthesis, the in situ generation of CO from CO 2 is clearly underdeveloped. Nevertheless, this strategy represents a particularly promising tool for more practical applications. We are convinced that such CO 2 valorization approach will open up new opportunities to realize industrially important carbonylation reactions. Advantageously, here CO 2 is used as a sustainable carbonyl source instead of hazardous CO. For more than 60 years, carbonylation reactions using CO represent major technology for the production of value-added bulk and fine chemicals from easily available feedstocks. As an example, over 10 million tons of oxo-products are produced every year from alkenes via hydroformylation and related tandem reactions [78] . Besides, methyl propionate, a key intermediate for methyl methacrylate (annual demand is currently about 3 million tons), is in part produced by palladium-catalysed methoxycarbonylation of ethylene [79] . So far, all these processes make use of CO, which is also difficult to transport on a bulk scale. Notably, the physical properties of carbon monoxide (especially its toxicity) impede its wider use in academia too. In this respect, carbonylations with CO 2 offer a more safe and accessible tool for synthetic organic chemists. The general strategy to use carbon dioxide as a carbonyl source is based on the in situ reduction of CO 2 to CO, which then can be used in subsequent carbonylation reactions. It is long known that combination of carbon dioxide and H 2 at high temperature (>300 °C) allows for so-called reverse water gas shift (RWGS) reaction, in which a mixture of carbon monoxide, carbon dioxide, hydrogen and water is formed. On the basis of their previous studies on the RWGS process, Tominaga and Sasaki et al. [80] reported in 2000 the first ruthenium-catalysed hydroformylation/reduction of alkenes with CO 2 using Ru 3 (CO) 12 as catalyst in the presence of LiCl as additive. It is surprising that this seminal work of Tominaga et al. has attracted only minor attention, probably due to the still drastic conditions and the efficiency of the reaction. For example, unwanted alkene hydrogenation side reactions occurred. Recently, our group improved this process by the application of a specific bulky phosphite ligand ( Fig. 7a ) [81] . Applying the optimized catalytic system, the yields of alcohols, the chemoselectivity of the process and especially the TON of the catalyst was significantly improved compared with the known ligand-free catalysis system. In the above-mentioned carbonylation reactions via RWSG reaction, water is always produced as a side product and is not involved in the following alkene carbonylation reactions. Remarkably, the group of Leitner [82] reported a rhodium-catalysed hydrocarboxylation of alkenes with CO 2 and H 2 to produce carboxylic acids, in which in situ -formed H 2 O was utilized as the nucleophile in this transformation ( Fig. 7b ). 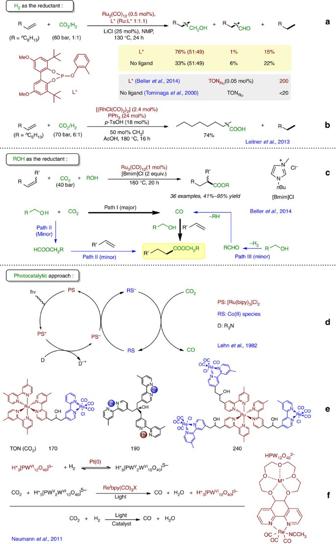Figure 7: Catalytic production of CO from CO2reduction and its application in carbonylation reactions. (a,b) H2as the reductant. (c) Alcohol as the reductant. (d–f) Photocatalytic approach. Figure 7: Catalytic production of CO from CO 2 reduction and its application in carbonylation reactions. ( a , b ) H 2 as the reductant. ( c ) Alcohol as the reductant. ( d – f ) Photocatalytic approach. Full size image Although H 2 can act as an efficient reducing reagent for CO 2 reduction, in many cases the following carbonylation reaction does not tolerate H 2 due to the hydrogenation of the substrate. As a result, the development of other benign CO 2 reductions to generate CO is highly desired for the valorization of CO 2 . Combining our long-term experience in alcohol dehydrogenation [83] and carbon dioxide reduction reactions [5] , [84] , very recently efficient reforming processes of alcohols and CO 2 were developed. This allows for catalytic alkoxycarbonylation reactions using CO 2 as the C1 source in the presence of a ruthenium/[Bmim]Cl catalyst system. Key to success was an unprecedented in situ formation of CO from CO 2 ( Fig. 7c ) [85] . In contrast to previously reported hydrocarboxylation reactions of alkenes with CO 2 , similar carboxylated products are obtained, but the presence of stoichiometric amounts of strong and expensive reductants like Et 2 Zn and silanes is avoided. The following reaction steps are proposed: initially, CO 2 is reduced to CO (path I) or alkyl formates (path II) through transfer hydrogenation with alcohols. Path I is proposed to be the major reaction pathway for this transformation based on the control experiments. Meanwhile, the alcohol undergoes dehydrogenation to form the corresponding carbonyl compound (path III). Interestingly, a minor amount of the CO comes from further decarbonylation reactions of the alcohol as shown by isotope-labelling experiments. It is estimated that this novel methodology is applicable to other carbonylation reactions as well and will contribute substantially to the development of next-generation CO 2 utilization. Apart from CO 2 reduction with hydrogen and alcohols, Skrydstrup and co-workers shortly afterwards reported the successful identification of an efficient conversion of CO 2 to CO performed at room temperature with catalytic caesium fluoride in the presence of a disilane, which can be coupled to Pd-catalysed amino- and alkoxycarbonylations with aryl bromides and iodides [86] . Inspired by nature’s efficiency in converting carbon dioxide into carbohydrates and other organic matter through photosynthesis, chemists have also explored opportunities to directly reduce CO 2 to CO by photocatalytic means. Since CO 2 does not absorb either visible or ultraviolet radiation in the wavelengths of 200–700 nm, this process requires a suitable photocatalyst to absorb ultraviolet–visible radiation and transfer it to CO 2 . Photosensitizers (PSs) that meet this criterion often include a metal centre, as the d -orbital splitting in organometallic species often falls within the energy range of far-ultraviolet and visible light. The reduction process begins with excitation of the PS. This causes the transfer of an electron from the metal centre into the coordinated ligands. This movement is termed as metal-to-ligand charge transfer process. Back-electron transfer from the ligands to the metal after the charge transfer is prevented by including an electron-donating species to quench the exciting state of the photocatalyst, thus forming the one-electron-reduced (OER) intermediate for further CO 2 reduction processes [87] . Initial work by Lehn and co-workers in the 1980s led the development of first photocatalytic CO 2 reductions. Here, CoCl 2 was used as the catalytic site for CO 2 reduction with [Ru(bpy) 3 ]Cl 2 as PS ( Fig. 7d ) [88] . However, CoCl 2 has very low selectivity towards the reduction of CO 2 to CO, resulting from the reduction of water in the aqueous media to produce H 2 that is the main product in this system. The TON of (CO+H 2 ) is only 32 based on [Ru(bpy) 3 ]Cl 2 . The efficiency of these photocatalytic processes is also characterized by its quantum yield Ф, which is defined as the number of times a CO 2 molecule is transformed per photon absorbed by the PS. However, this system reached a quantum yield of only 1.2%. Despite the low selectivity and efficiency of this reaction, the simultaneous reduction of CO 2 and H 2 O produces in fact syngas, which is of interest for large-scale industrial processes. Moreover, it represents an early step in the development of chemical systems capable of artificial photosynthesis and solar energy conversion. Later, the same research group found that rhenium-based complexes [Re(bipy)(CO) 3 X] (X=Cl, Br) acting as both PS and catalyst are more efficient and represent more selective catalysts for CO 2 reduction [89] . The process has very high CO/H 2 , selectivity, generating only CO, and affords a quantum yield of up to 14%. It is indicated that the dissociation of the ligand X − from the unstable 19-electron OER is a key step in this photocatalytic reduction of CO 2 (ref. 90 ). In addition, Fujita and co-workers identified the binuclear [Re-C(O)O-Re] moiety as a key intermediate of the two-electron reduction process from CO 2 to CO (ref. 91 ). In 2008, based on their insightful mechanistic study, the most efficient photocatalytic system was successfully developed by the group of Ishitani using a mixed catalysts’ system with fac -[Re(bpy)(CO) 3 (CH 3 CN)] + and fac -[Re-4,4′-(MeO) 2 bpy(CO) 3 P(OEt) 3 ] + affording the optimized quantum yield for CO formation was 0.59 (ref. 92 ). Despite the improved activity of rhenium polypyridine complexes for CO 2 reduction, a major problem with these photocatalysts is the lack of an extended absorption into the visible region. To solve this problem, Ishitani and Bian and co-workers presented the use of covalently linked heteronuclear Ru and Re multimetallic complexes in the photocatalytic reduction of CO 2 (refs 93 , 94 ). Enhancement of the photocatalytic response to light in the visible region was achieved by specifically designed supramolecular complexes, and their high photocatalytic activities were attributed to intramolecular electron transfer from the OER Ru species to the Re moiety. The binuclear complex Ru–Re, trinuclear complex RuRe 2 and tetranuclear complex RuRe 3 all furnished higher TON of CO ( Fig. 7e ). Despite recent improvements [95] , it should be noted that, in the above-mentioned photochemical CO 2 reduction, common sacrificial donors such as triethylamine (TEA), triethanolamine (TEOA) and 1-benzyl-1,4-dihydronicotinamide (BNAH) have to be used. From a practical point of view, it is noteworthy that in 2011 Neumann and co-workers [96] developed a photoreduction of CO 2 to CO with H 2 catalysed by a rhenium(I) phenanthroline-polyoxometalate hybrid complex. In this study, previously used sacrificial electron donors were replaced by H 2 . The working catalysis system is summarized in Fig. 7f . On one hand, a polyoxometalate oxidizes H 2 to two protons and two electrons in the presence of Pt(0). On the other hand, the reduced form of the polyoxometalate reacts with CO 2 with the assistance of a chromophoric rhenium(I) complex and visible light to produce CO and H 2 O. As a result, the overall reaction is a photocatalytic RWGS reaction, which is of interest for both industry and academia for its further potential application in carbonylation reaction with CO 2 . Today’s chemical production as well as academic organic synthesis relies mainly on the use of fossil-based carbon sources. In contrast, the increased valorization of CO 2 as a recyclable and abundant C1 building block would allow for the development of a sustainable chemical industry. In this respect, the development of benign transformations of carbon dioxide is a highly attractive object for synthetic chemistry. Clearly, in the past decades, several effective activation modes for catalytic CO 2 fixation and a series of novel transformations have been disclosed. Issues need to be resolved Despite the impressive progress, the efficiency of most reactions is far from satisfying. Hence, only recent new processes utilizing CO 2 as the C1 source have been industrialized. In most methodology-driven work, there remain important issues that need to be addressed in the future, for example, less utilization of very reactive/sensitive reagents, extending substrate scope, milder reaction conditions, improved chemo- and regioselectivity. Due its inherent inertness, not surprisingly, reactions of carbon dioxide under mild conditions need a thermodynamic driving force, for example, energy-rich coupling partners. The copolymerization of epoxides with CO 2 to produce polycarbonates is an elegant example for this strategy and permits efficient CO 2 valorization. Alternative copolymerizations with easily available chemical feedstocks, such as olefins, are highly desired too. In this respect, the recent report from Nozaki’s group of a copolymerization of CO 2 and 1,3-butadiene is interesting. This work provides a straightforward approach towards the production of novel polymeric materials from CO 2 (ref. 97 ). Another promising field might be the use of carbon dioxide as methylation agent. For example, ruthenium-catalysed methylation of amines with CO 2 and H 2 to afford valuable products has very recently been achieved. However, the current catalyst loading is still too high for large-scale production. Hence, the development of more efficient catalyst systems and non-noble metal-based catalysts for this and related transformations constitutes a demanding goal. Most of the CO 2 -fixation reactions, which proceed via oxidative cyclometallation pathway, are restricted to extensive π systems (dienes and diynes) as substrates and the use of zinc reagents to cleave the metallacycle intermediates. Consequently, utilization of other simple alkene or alkyne substrates and milder nucleophiles is highly desired to further improve this strategy. Carboxylation reactions via CO 2 insertion into C-M bonds in combination with classical coupling reactions are intensively studied in the past 10 years. Although this strategy furnished a series of interesting transformations, the requirement of stoichiometric amounts of strong bases, sensitive metal reagents or expensive hydrosilanes are evident drawbacks that need to be overcome. The key point to solve such problems in the future will be the invention of new routes to quench metal carboxylate complex (RCOOM) with less-nucleophilic agents to afford the final product and regenerate the original catalytically active species. Finally, it is worth noting that the catalytic in situ generation of CO from CO 2 and its recent applications in sequential carbonylation reactions is a more favourable strategy for CO 2 valorization. It provides the use of safe and abundant CO 2 instead of CO as carbonyl source. Here the improvement of (regio)selectivities and to use milder reaction conditions represent important targets. So far, most catalysts in such reactions are ruthenium-based complexes. Encouraged by the recently developed highly regioselective ruthenium-catalysed hydroformylation reaction [98] , [99] , in the future more efforts should be donated to solve the regioselectivity problem with suitable ligands and/or additives. Last but not the least, similar to other catalysis processes, the discovery of non-noble metal-catalysed reactions, for example, iron catalysts, is an essential issue in this field. Although related photocatalytic approaches proceed under very mild conditions, the TON is too low currently. Probably, cascade reaction sequences that make use of carbonylation processes to consume the in situ -generated CO will drive the overall reaction more efficiently. Towards artificial photosynthesis Photosynthesis basically supplies the carbon source for all organic compounds on Earth. It is an ideal green process for the conversion of light energy into chemical energy, which makes use of CO 2 ( Fig. 8 , equation a). Inspired by the nature’s strategy, the development of sustainable and straightforward catalytic C-C bond-forming reactions of CO 2 in industrially relevant target molecules will be the ‘crown jewel’ of organic synthesis and catalysis research in the future. We expect several dream reactions towards artificial photosynthesis (CO 2 reduction under very mild conditions) and beyond will become true in the coming years. For example, sodium acrylate is an industrially important acrylate, with a global market volume of about 4 million tons and is commonly used as a monomer in the production of superabsorber polymers. Thus, the direct synthesis of acrylic acid from CO 2 and ethylene represents an economically attractive but also most challenging dream reaction. Until now, a TON of only 10 (Ni catalyst and NaO t Bu as base) has been realized; nevertheless, the possibility of this reaction was clearly demonstrated ( Fig. 8 , equation b) [100] . Ethylene glycol is another important raw material in the manufacture of polyester fibres and polyethylene terephthalate resins used in bottling. The direct hydrogenation of CO 2 to produce this chemical in bulk scale might be a prime example for selective reductive coupling using carbon dioxide and could substitute its traditional synthesis from ethylene oxide ( Fig. 8 , equation c). As a final example, the reductive methylation of more widely available arenes, for example, benzene (from biogas), to generate toluene and xylenes is also highly interesting ( Fig. 8 , equation d). 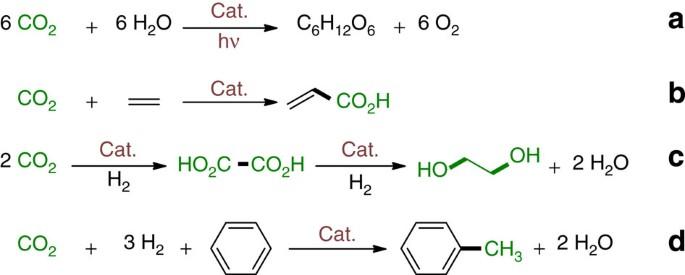Figure 8: Dream reactions towards artificial photosynthesis. (a) Photosynthesis reaction process. (b) Direct synthesis of acrylic acid from ethylene and CO2. (c) Ethylene glycol synthesis via reductive coupling of CO2. (d) Reductive methylation of benzene using H2and CO2. Figure 8: Dream reactions towards artificial photosynthesis. ( a ) Photosynthesis reaction process. ( b ) Direct synthesis of acrylic acid from ethylene and CO 2 . ( c ) Ethylene glycol synthesis via reductive coupling of CO 2 . ( d ) Reductive methylation of benzene using H 2 and CO 2 . Full size image Above all, it is anticipated that more research groups will join this very promising but also challenging field to discover a number of applied organic synthesis approaches using CO 2 as the C1 building block, in which the employment of less-active substrates, reduced waste generation and milder reaction conditions should be addressed. How to cite this article : Liu, Q. et al. Using carbon dioxide as a building block in organic synthesis. Nat. Commun. 6:5933 doi: 10.1038/ncomms6933 (2015).